B-cell depletion reveals a role for antibodies in the control of chronic HIV-1 infection HIV can be partially contained by host immunity and understanding the basis of this may inform vaccine design. The importance of B-cell function in long-term control is poorly understood. One method of investigating this is in vivo cellular depletion. In this study, we take advantage of a unique opportunity to investigate the role of B cells in an HIV-infected patient. The HIV-1 + patient studied here was not taking antiretroviral drugs and was treated for pre-existing low-grade lymphoplasmacytoid lymphoma by depletion of CD20+ B cells using rituximab. We demonstrate that B-cell depletion results in a decline in autologous neutralizing antibody (NAb) responses and a 1.7 log 10 rise in HIV-1 plasma viral load (pVL). The recovery of NAbs results in a decline in pVL. The HIV-1 sequences diversify and NAb-resistant mutants are subsequently selected. These data suggest that B-cell function can contribute to the long-term control of pVL, and that NAbs may be more important in controlling chronic HIV-1 infection than previously suspected. HIV-1 is readily able to evade host defence and establish persistent infection. The virus may, however, be partially contained by host adaptive immunity, including both B- and T-cell responses. There is good evidence that CD8+ T-cell responses have a role in viral suppression. For example, there are strong HLA class I associations with clinical outcome [1] , and in the SIV model, macaques in whom CD8+ T cells are depleted show significant increases in their viral load [2] . These findings have led to a major initiative to develop T-cell-based vaccines, and much work to define the correlates of protection based on assays of T-cell function [3] , [4] . However, as a leading HIV vaccine candidate failed to induce protective T-cell responses [5] and recent trial data suggest partial protection from a vaccine including a gp120 component [6] , the incentive to understand the role of neutralizing antibodies (NAbs) and of B cells in HIV infection has increased considerably [7] , [8] , [9] . B cells have a multifaceted role in humoral and cellular responses to HIV-1, yet their impact in containing the virus remains unclear. This is partly because of the complex nature of the antigenic target (gp120) [10] . Key obstacles to the development of both T- and B-cell defence are the abilities of the HIV-1 genome to integrate and also evolve rapidly in the face of immune selection pressure: the latter feature results from both the high replication rate of the virus and the error-prone nature of the HIV-1 reverse transcriptase, which lacks proofreading capacity [11] . These mutations are readily accommodated within gp120 because of plasticity of the structure and the capacity to acquire glycosylation sequons that provide a 'glycan shield' [12] . Therefore, emerging NAbs repeatedly select mutant viruses that are resistant to neutralization [13] . The NAb response also evolves through somatic recombination and affinity maturation of proliferating B cells, but is only partially effective against concurrently circulating viruses, while retaining potent activity against strains previously circulating within the patient [13] , [14] , [15] . Such data have cast doubt on the contribution of NAbs to the control of virus load, despite the counterargument that NAbs must inhibit virus replication to drive the selection of resistant variants. Monoclonal antibodies have been identified that both cross-recognize and potently neutralize a variety of HIV-1 strains [16] , [17] , [18] , [19] . The targets for these are well defined and include, among others, CD4 and co-receptor binding sites and epitopes within the gp41 fusion subunit [20] . These areas are under some structural constraint compared with other epitopes, such as in the exposed variable loops. Few potent monoclonal antibodies have been isolated, yet the proportion of gp120-specific antibodies capable of neutralization may be greater than once believed [8] , [21] . Recent studies indicate that some individuals possess NAbs that exhibit broad and potent neutralization capacity [18] , [21] , [22] , but functional data to causally link such antibodies to the control of viremia are lacking. Furthermore, the contribution of B-cell responses to the containment of plasma viral load (pVL) has been difficult to determine, because of other important factors that limit virus replication, such as T-cell response, virus fitness and host genetics [23] . Historically, functional importance has been confidently attributed to specific arms of the immune response by means of experiments that deplete or transfer that effector arm. Although such data are readily available in animal models, they are rarely available in humans. As recent vaccine studies have highlighted substantial differences between SIV models and HIV, it is important to seek such evidence in human studies. Rituximab (Rituxan, MabThera; Roche) is a monoclonal antibody targeting CD20 antigen expressed on most B cells, with the exception of the terminally differentiated plasma cells. It has become widely used for treatment of lymphoma and also of antibody-mediated autoimmune diseases [24] . We report a unique case in which rituximab monotherapy was used in a patient with stable viraemia, in the absence of antiretroviral therapy (ART). By combined analyses of viral dynamics, viral evolution and autologous NAb responses, we show reversible loss of HIV-1 control following rituximab monotherapy. Loss of control was associated with reduction in titres of NAbs targeting the CD4 binding site, as well as with an increase in genetic diversity and transient reversion to NAb-sensitive virus. As NAb levels later increased, pVL was once more controlled and this was accompanied by further immune selection of NAb-resistant viruses. These data suggest that despite ongoing immune escape, NAbs secreted by CD20+ B cells may have a significant role in control of pVL during chronic HIV-1 infection, a finding of significance for HIV-1 immunotherapies and vaccines. Clinical course of the study subject The patient, a Caucasian man, was diagnosed with HIV seroconversion illness at the age of 58 years. Three years earlier, he was diagnosed with low-grade lymphoplasmacytoid lymphoma, for which he did not receive treatment [25] . Histologically, this was defined as a small lymphocytic B-cell lymphoma with plasmacytoid differentiation mostly expressing CD20 and CD79. The tumour was IgM secreting. His only other medical history of note was an acute hepatitis B infection approximately 30 years earlier. Following HIV-1 seroconversion, the patient was recruited into a prospective, non-randomized observational study of early treatment and received 3 months of highly active antiretroviral therapy [26] . After 30 months, he developed a rising paraproteinaemia, attributed to his lymphoma, and received thalidomide treatment without clinical effect. He initiated rituximab therapy 1,075 days after HIV seroconversion and received four weekly doses (375 mg m −2 ). He felt unwell 20 weeks after the first dose of rituximab with malaise and fever associated with a marked rise in HIV pVL (increase of 1.7 log 10 ; Fig. 1 ). In addition, he developed biochemical hepatitis (attributed to reactivation of hepatitis B) that resolved with only supportive treatment. Antiretrovirals were initiated 1,392 days after seroconversion. 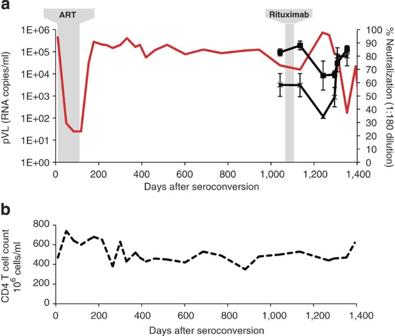Figure 1: Autologous neutralizing antibody titres over time. (a) Pseudotyped virus particles were constructed using full-length envelope clones that represent majority quasi-species at 336 or 1,042 days after seroconversion. Plasma VL over time is indicated (red line). The brief dip in viral load over the first 100 days represents the period of initial ART as part of the short-course ART trial (shaded grey). The neutralizing effects (%; rightyaxis) of patient sera are shown for autologous viruses constructed with clonedenvgenes derived 336 days (black squares) and 1,042 days (crosses) after seroconversion. Results from a single clone (tested in triplicate) representative of three clones are shown. Serum was sampled sequentially before and after rituximab therapy (1,075–1,106 days, shaded grey), and assayed at concentrations ranging from 1:20 to 1:4,370; the neutralizing effects of sera diluted 1:180 are shown here. Error bars show standard deviations of triplicate tests. (b) CD4 T lymphocyte count (dashed line) is shown over time. Figure 1: Autologous neutralizing antibody titres over time. ( a ) Pseudotyped virus particles were constructed using full-length envelope clones that represent majority quasi-species at 336 or 1,042 days after seroconversion. Plasma VL over time is indicated (red line). The brief dip in viral load over the first 100 days represents the period of initial ART as part of the short-course ART trial (shaded grey). The neutralizing effects (%; right y axis) of patient sera are shown for autologous viruses constructed with cloned env genes derived 336 days (black squares) and 1,042 days (crosses) after seroconversion. Results from a single clone (tested in triplicate) representative of three clones are shown. Serum was sampled sequentially before and after rituximab therapy (1,075–1,106 days, shaded grey), and assayed at concentrations ranging from 1:20 to 1:4,370; the neutralizing effects of sera diluted 1:180 are shown here. Error bars show standard deviations of triplicate tests. ( b ) CD4 T lymphocyte count (dashed line) is shown over time. Full size image Impact of B-cell depletion on NAb titres Following rituximab therapy, the subject's HIV-1 pVL, previously stable, increased by more than 1.7 log 10 , peaking at 737,400 copies per ml 4 months after the final dose of rituximab ( Fig. 1 ). The pVL subsequently returned to baseline levels in the absence of ART. We therefore analysed the impact of rituximab therapy on NAb titres in relation to viral dynamics. Rituximab therapy led to a 30% reduction in total IgG levels, which reached their lowest point at the peak of virus load (10.8 g l −1 ; normal range 8–16 g l −1 ) and returned to pre-rituximab levels thereafter ( Supplementary Table S1 ). To evaluate NAb activity throughout this period, we generated pseudoviruses derived from autologous envelope ( env ) sequences. Serum obtained before the first dose of rituximab potently neutralized virus pseudotyped with autologous envelope derived from plasma acquired 2 years previously (day 336 after seroconversion) ( Table 1 ). The same serum neutralized contemporaneous autologous Env pseudotypes, although to a lesser extent, with 1:60 serum dilutions effectively blocking more than 90% infection. 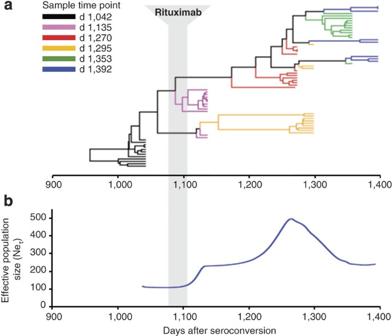Figure 2: Diversification of HIV-1envsequences after rituximab therapy. (a) A time-structured tree, showing divergence-time estimates among intra-host plasma HIV-1 clonal sequences before and after rituximab therapy (shaded grey), based on a Bayesian relaxed molecular clock applied to 969 nucleotides58. The external nodes represent sequences taken from time points indicated by the colours given in the figure key (inset). The topology is of the highest likelihood calculated using BEAST, with branch lengths proportional to time estimates for the subtending nodes (summarizing 60 million Markov chain Monte Carlo (MCMC) simulations, generated after discarding 6 million as burn-in). All the parameters in the MCMC started from random values, except for substitution rates and population size, where the priors were imported from the combined proviral and plasma viral sequence data of the same host calculated by BEAST software. (b) The effective population sizes (Neτ) were calculated using BEAST. Thexaxis (days after seroconversion) is the same as forFigure 2a59. Heterologous NAb activity was also observed against HXB2 and 8/12 Tier 2/3 clade-B reference strains (NIH, AIDS) ( Table 2 ). Following rituximab therapy, we observed a marked decrease in neutralizing activity characterized by a drop of more than threefold in IC 50 serum titres against day 336 Env pseudotypes, which recovered over a 4-month period. Strikingly, these changes coincided with the increase in pVL. Recovery of NAb responses correlated with control of viraemia ( Fig. 1 ). Table 1 IC 50 neutralizing titres against autologous viruses. Full size table Table 2 IC 50 neutralizing titres against heterologous viruses. Full size table Analysis of sequence evolution in HIV-1 envelope over time To evaluate sequence evolution over this period, env products were generated by reverse transcription (RT)–PCR from plasma viral RNA, before and after rituximab therapy (days 1,075–1,392; Fig. 2a ). We identified clear sequence diversification as the virus peaked during rituximab treatment (mean genetic distance=0.02 versus 0.004; P <0.0001). This diversification manifested as an increase in effective population size as measured using BEAST [27] (fivefold change; Fig. 2b ). To assess whether these diverse strains represented a re-emergence of archived provirus, we used an identical sequencing strategy to analyse stored peripheral blood mononuclear cell (PBMC) samples available from the time of seroconversion up to day 1,042; these sequences were placed on a time-structured tree ( Supplementary Fig. S1 ). Viruses detected after rituximab treatment did not represent re-emergence of early archived strains; those strains present as pVL peaked were most closely related to strains present in plasma at day 1,042, with a subset related to those archived in PBMC at day 1,042. Figure 2: Diversification of HIV-1 env sequences after rituximab therapy. ( a ) A time-structured tree, showing divergence-time estimates among intra-host plasma HIV-1 clonal sequences before and after rituximab therapy (shaded grey), based on a Bayesian relaxed molecular clock applied to 969 nucleotides [58] . The external nodes represent sequences taken from time points indicated by the colours given in the figure key (inset). The topology is of the highest likelihood calculated using BEAST, with branch lengths proportional to time estimates for the subtending nodes (summarizing 60 million Markov chain Monte Carlo (MCMC) simulations, generated after discarding 6 million as burn-in). All the parameters in the MCMC started from random values, except for substitution rates and population size, where the priors were imported from the combined proviral and plasma viral sequence data of the same host calculated by BEAST software. ( b ) The effective population sizes (Ne τ ) were calculated using BEAST. The x axis (days after seroconversion) is the same as for Figure 2a [59] . Full size image Immune selection and neutralization of HIV-1 envelope The apparent in vivo impact of the NAbs in this individual prompted a search for the targets of binding. To identify potential NAb targets, we first analysed immune selection using CODEML, analysing the ratio of non-synonymous to synonymous mutations (d N /d S ) at each site. We observed two sites under selection ( Fig. 3 ; Supplementary Fig. S1 )—position 339 (d N /d S =7.6, P <0.0001) and position 363 (d N /d S =6.977, P =0.03). Residue 363 lies between the β14 and β15 anti-parallel strands of gp120 and is exposed on the surface of the outer domain in close proximity to the CD4 binding loop [28] . Computational modelling of atomic level envelope structures has shown that mutations proximal to the CD4-binding loop are critical in conferring resistance to CD4bs antibodies [29] . Furthermore, site-directed mutagenesis of site 363 has previously been shown to affect neutralization of the CD4bs antibodies M-14 and b12 [30] , [31] . Before the first dose of rituximab (day 1,042 after seroconversion), position 363 was occupied by an arginine in all viral RNA sequences, whereas all proviral DNA clones sampled up to and including day 1,042 had a glutamine at the same position. Following rituximab therapy, R363 variants were temporarily replaced with Q363 variants, which reverted to arginine residues as NAb titres rebounded and viraemia was controlled. 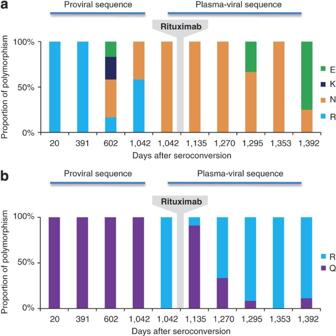Figure 3: Tracking of selected envelope mutants. This figure shows the relative frequencies of polymorphisms at sites (a) 339, dN/dS=7.61P<0.0001 and (b) 363 dN/dS=6.98P<0.031. The individual bars along thexaxis represent the different time points of sequencing (comparable toFig. 2;Supplementary Fig. S1): these are taken either from proviral DNA samples (days 20–1,042) or from plasma samples (days 1,042–1,392). The time of rituximab therapy is indicated. Each bar shows the frequency of mutations at these positions, the key depicts the different amino-acid residues detected. Figure 3: Tracking of selected envelope mutants. This figure shows the relative frequencies of polymorphisms at sites ( a ) 339, d N /d S =7.61 P <0.0001 and ( b ) 363 d N /d S =6.98 P <0.031. The individual bars along the x axis represent the different time points of sequencing (comparable to Fig. 2 ; Supplementary Fig. S1 ): these are taken either from proviral DNA samples (days 20–1,042) or from plasma samples (days 1,042–1,392). The time of rituximab therapy is indicated. Each bar shows the frequency of mutations at these positions, the key depicts the different amino-acid residues detected. Full size image Before rituximab therapy, an asparagine at site 339 formed part of an N -linked glycosylation site. This residue is located within the α3 helix, which is exposed on the surface of the protein according to atomic level structures. A previous study showed that site 339 is involved in recognition by 2G12, a monoclonal antibody the binding of which is carbohydrate dependent [32] . However, in addition to this, mutations at site 339 have been reported to affect binding by monoclonal antibody b12: this effect is observed despite site 339 being some distance away from the CD4 binding site, and potentially occurs through conformational perturbation [32] . No other sites in the envelope were found to be under positive selection, indicating that mutations at these positions affected NAb binding. To examine the effect of sequence changes on neutralization susceptibility, pseudoviruses mimicking Q363R and R339N/E were constructed by site-directed mutagenesis. The selected Q363/339E mutation reduced the IC 50 titres of day 1,042 serum by more than twofold (IC 50 from >775 to 300). Confirming previous data, the Q363R mutation was also shown to inhibit neutralization by fivefold by antibody b12 [31] whereas N339E inhibited neutralization susceptibility by fourfold to the carbohydrate-specific antibody 2G12 [12] , [32] . To further define the site of binding of the patient's NAbs, we performed a direct competition experiment using well-defined monoclonal antibodies and recombinant clade B envelope as the antigenic target ( Fig. 4 ). This experiment showed strong binding competition between patient sera and antibodies b12, 4.8d (which targets an epitope overlapping with the co-receptor binding site) and 447-52D (which targets the V3 loop). No competition was observed against 2G12. The experiment also revealed a clear decline in competition for binding in samples taken during the peak of viraemia, which recovered as pVL declined, in good accordance with the data obtained from the neutralization experiments, but using an independent system of evaluation ( Fig. 4b ). 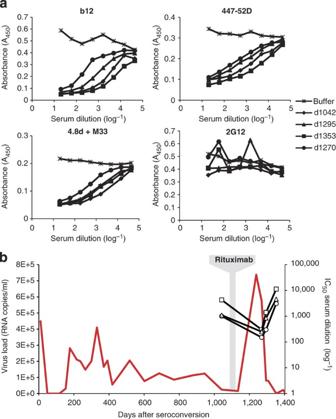Figure 4: Characterization of patient antibodies by competition ELISA. (a) Serial dilutions of patient serum (xaxes) collected on days 1,042 (filled diamonds), 1,270 (filled circles), 1,295 (filled triangles) and 1,353 (filled squares) after seroconversion reduced gp120 binding with NAbs b12, 447-52D and 4.8d, thereby reducing colorimetric change and light absorption (A450 nm,yaxes). Pooled serum collected from HIV-uninfected subjects (stars) did not compete with any NAb for gp120 binding. All sera failed to compete with 2G12 for gp120 binding. (b) The reciprocal dilutions of sera, sampled before and after rituximab therapy, which reduce gp120-NAb binding by 50% (IC50, rightyaxis). Hundred percent binding was taken as that observed in microtitre wells containing IgGb12 (empty squares), 4.8d (empty triangles) or 447D (empty circles) in the absence of patient sera. Corresponding VLs are shown by the red line (leftyaxis). Figure 4: Characterization of patient antibodies by competition ELISA. ( a ) Serial dilutions of patient serum ( x axes) collected on days 1,042 (filled diamonds), 1,270 (filled circles), 1,295 (filled triangles) and 1,353 (filled squares) after seroconversion reduced gp120 binding with NAbs b12, 447-52D and 4.8d, thereby reducing colorimetric change and light absorption (A 450 nm , y axes). Pooled serum collected from HIV-uninfected subjects (stars) did not compete with any NAb for gp120 binding. All sera failed to compete with 2G12 for gp120 binding. ( b ) The reciprocal dilutions of sera, sampled before and after rituximab therapy, which reduce gp120-NAb binding by 50% (IC 50 , right y axis). Hundred percent binding was taken as that observed in microtitre wells containing IgGb12 (empty squares), 4.8d (empty triangles) or 447D (empty circles) in the absence of patient sera. Corresponding VLs are shown by the red line (left y axis). Full size image Analysis of other potential effects of rituximab We investigated other possible causes for the observations made, particularly the possibility of an indirect impact on cellular immunity [33] . We analysed the sequence of key CTL epitopes over time, and carried out interferon-γ (IFN-γ) ELISpot analyses. Although some mutations in pre-rituximab sequences were observed, the majority of the epitopes remained stable ( Table 3 ). It is of importance that control over pVL was regained without further escape/reversion at these sites. Table 3 Analysis of CD8+ T cell responses and epitope evolution over time. Full size table Second, immune activation through recrudescence of other infectious agents may have a role in this case. Concurrent with the pVL increase, the patient also developed elevated liver transaminases, associated with reactivation of previously controlled hepatitis B virus (HBV) infection [34] . However, control of HIV was observed at a time when HBV load was still high, suggesting that HBV replication per se was not driving HIV replication (up to day 1,389; Supplementary Fig. S2 ) in this patient. In the setting of acute illness, there was no evidence of EBV, HHV-6, HHV-8 or HCV in blood. Cytomegalovirus was present only at low copy number (50 copies per ml). A bronchoalveolar lavage was tested for a broad panel of relevant viruses, all of which were negative, including VZV and HSV1/2. Clearly, these data do not exclude reactivation of a further latent infection, or concurrent superinfection, although the major herpesvirus infections appear unlikely to be contributing significantly. In this study, B-cell depletion led to a decline in NAb titres against HIV, concurrent with rising pVL. Recovery of NAb titres coincided with control over viral load. Multiple analytical techniques were used to longitudinally characterize the distinct virus population that emerged as NAbs returned. The common ancestor of this new virus population was defined by polymorphisms at two residues exposed on the surface of the virus envelope, both of which showed evidence of positive selection, with mutations affecting binding of NAbs. There are no published studies on the impact of rituximab alone on HIV viraemia in humans. Studies on acute SIV mac infection in macaques treated with rituximab indicate a role for NAb responses in containing post-acute viral load [35] , [36] . In contrast, a recent study using African Green monkeys did not reveal any effect of rituximab treatment during acute SIV agm infection [37] ; thus, data from human studies are important to resolve this issue. It is possible that depletion of B cells had an indirect impact on viral load through modulation of CD4+ or CD8+ T-cell subsets. Although we cannot exclude this, the mechanism for such an indirect effect is not clear and, importantly, no impact on CD8+ T-cell responses has been observed in the SIV models quoted above [36] . The delay of several weeks that is observed between rituximab treatment and the change in viral load is much more consistent with the observed decline in antibody titres than a direct B-cell/T-cell interaction, which would be expected to take effect immediately. In addition, the changes in the prevailing sequence (reversion and subsequent re-selection of a mutated NAb epitope; Figs 2 , 3 ; Supplementary Fig. S1 ) are consistent with relaxation and re-application of NAb-mediated selection pressure. The impact of other reactivating viruses on HIV load is complex. As in this case, rituximab treatment is known to have the potential to reactivate HBV [38] , even in those with previously controlled infection (HbsAg−, HBcoreAb+). This points to an important role for B cells in long-term control of HBV—a virus in which CD8+ T cells have an important role in acute disease [39] . The relationship between HBV pVL and HIV pVL is not fully understood, but overall these appear to be independent [40] , [41] . In this case, HBV and HIV pVL increased within a similar timeframe; however, control over HIV occurred spontaneously, whereas HBV load remained high, indicating that they were differentially regulated in this patient ( Supplementary Fig. S2 ). However, this does not exclude a secondary impact of HBV through induction of liver inflammation or other consequences of immune activation. In addition, although we did not find other evidence of systemic reactivation of other major pathogens in this individual, it remains possible that local or low-level reactivation could also affect HIV pVL. Overall, our findings support previous suggestions of an evolutionary balance between virus and NAbs [12] , [42] . At first sight, these findings appear at odds with previous studies that fail to confirm an association between long-term virus control and NAb response, especially in elite controllers [43] . However, as shown here, the dynamics of immune responses are critical to their interpretation; therefore complex relationships could easily be missed in cross-sectional studies, especially analyses of those with favourable CD8+ T-cell responses [1] , [43] , [44] . There is a clear relationship between the changes in NAb titre and pVL demonstrated in this study, although the mechanism of action of such NAbs in vivo may be complex. Studies using engineered antibodies in which Fc binding was disrupted have shown that interactions of NAbs with infected cells, leading to engagement of effector cells, may provide an important component of the protective capacity in vivo [45] , [46] . It is also possible that other non-NAb specificities not defined using in vitro NAb assays might have a role in vivo [47] . It is noteworthy that as B-cell responses to HIV envelope may be poorly sustained, it has been proposed that long-term plasma cell pools may not be established (reviewed in refs 48 , 49 ). As plasma cells are spared the effects of rituximab [50] (and total IgG levels therefore remain relatively less affected), it is suggested that the antiviral NAbs identified here, and potentially elsewhere, are maintained by B-cell populations that express CD20. In conclusion, this unique study suggests that B cells, and their secreted NAbs, can affect HIV viral load in chronic infection. This evidence, derived directly from observations in man, may inform the rational design of future immunotherapies and HIV vaccines. Construction of HIV-1 env expression cassettes The study was approved according to local ethical review (IRB Number 99/IA/161E). Full-length virus env was PCR amplified from cDNA obtained by RT of plasma-derived viral RNA collected 336 and 1,042 days after seroconversion for construction of pre-rituximab Env-pseudotyped virus. The latter time point represented virus present around the time of rituximab treatment. The primers used were env 1A (outer sense, 5′-CACCGGCTTAGGCATCTCCTATGGCAGGAAGAA3′), env 1M (outer antisense and RT, 5′-TAGCCCTTCCAGTCCCCCCTTTTCTTTTA-3′) [51] , env F1/2 (inner sense, 5′-GGGCTCGAGACCGGTGAGCAGAAGACAGTGGCAATG(±A)-3′) and env R1/2 (inner antisense, 5′-AAATCTAGAGGGCCCCCATTGCCACCCATBTTA(±TAGC)-3′). Bulk PCR products were restriction-cloned into pcDNA3.1 (Invitrogen) using sites Apa I and Xho I to result in pcDNA3.1. env , followed by sequencing. Of 20 genetically distinct clones that were most representative of the consensus sequence, 3 were selected for neutralization experiments. Site-directed mutagenesis Where stated, 100 ng pcDNA3.1. env was used as a template for PCR amplification using PfuUltraII Fusion HS (Stratagene) in the supplied buffer supplemented with 250 μM dNTPs and 3% dimethylsulphoxide. Mutagenesis primers contained restriction sites inserted by synonymous mutation (underlined): R339Nf (5′-ATTGTAACATTT CTCGAG TAGAATGGAATGACACCTTAA-3′), R339Nr (5′-TTAAGGTGTCATTCCATTCTA CTCGAG AAATGTTACAAT-3′), R339Ef (5′-ATTGTAACATT TCTAGA GTAGAATGGGAAGACACCTTAA-3′), R339Er (5′-TTAAGGTGTCTTCCCATTCTAC TCTAGA AATGTTACAAT-3′), Q363Rf (5′-TAAAACAATAATCTTTA ATCGAT CCTCAGGA-3′) and Q363Rr (5′-TCCTGAGG ATCGAT TAAAGATTATTGTTTTA-3′). After 18 amplification cycles (95 °C for 50 s, 60 °C for 50 s and 68 °C for 9 min), dam -methylated PCR templates were eliminated by Dpn I restriction digestion. Mutant clones were identified by restriction analysis and confirmed by nucleotide sequencing. Double mutants were constructed by sequential PCR amplifications. Construction and neutralization of Env-pseudotyped virus particles Autologous env clones and a heterologous panel of subtype-B reference strains [52] were co-transfected with the HIV-1 backbone nl4.3Δ env [53] into 293T-17 human epithelial kidney cells using Lipofectamine 2000 (Invitrogen). At 48 h following transfection, supernatants were collected by 0.45-μm filtration and stored at −150 °C before titration onto the HIV-permissive reporter cell line, TZM-bl, which stably expresses Escherichia coli β-galactosidase under regulatory control of a Tat-responsive HIV-1 long terminal repeat. Cells were fixed with glutaraldehyde (0.2%) and stained with X-gal substrate 48 h after infection. After staining, infected cells formed 'blue' focus-forming units, which were counted under light microscopy to determine the virus titre. Autologous Env-pseudotyped virus was confirmed to be R5 tropic by titration onto CD4 + CCR5 + and CD4 + CXCR4 + GHOST cell lines, which express green fluorescence protein in response to viral Tat. For neutralization experiments, pseudotyped virus was incubated for 1 h with a threefold dilution series of heat-inactivated serum, or with broadly specific NAbs (b12 or 2G12) [12] . After 48 h, fixed and stained cells were manually counted and neutralization was measured as the percentage reduction of focus-forming units relative to non-neutralized virus controls. Samples were prepared in triplicate microtitre wells and counts were verified by separate investigators (DB and ET). Competitive binding assays Antibody specificity was mapped using a competitive-binding enzyme-linked immunosorbent assay (ELISA). High-binding microtitre plates (Greiner) were coated overnight with recombinant Bal-strain gp120 and blocked with 2% milk powder to limit non-specific antibody binding. Each plate received threefold dilution series of patient sera and was incubated with 50% saturating titres of biotinylated NAbs (b12, 2G12, 447-52D). An additional plate was pre-incubated with the CD4 peptide mimic M33 before incubation with biotinylated NAb 4.8d [54] . Bound NAb was detected with streptavidin horseradish peroxidase and TMB chromogen substrate. Serum-mediated inhibition of NAb binding was determined as the percentage reduction in light absorbance (A 450 nm ) compared with wells that received dilution buffer (PBS 0.05% Tween 20, 1% bovine serum albumin) instead of serum. ELISpot for interferon-γ secreting CD8+ T cells This was performed using panels containing optimized HLA-matched peptides [55] . Fresh PBMCs were tested for T-cell responses using ex vivo Interferon-γ ELISpot assays. 96-well nitrocellulose plates (Millipore) were coated with 0.05 μg ml −1 recombinant anti-IFN-γ (Mabtech) in PBS overnight at 4 °C. Plates were then washed seven times with PBS and blocked with R10 for 2 h at 37 °C. PBMCs (2×10 5 ) were added to each well and then stimulated with peptide. The final concentration for peptide stimulation was 10 μg ml −1 and each peptide was tested in duplicate. Medium alone was used as a negative control and 1 μg ml −1 phytohemagglutinin was used as a positive control for all assays. The assay plates were incubated for 18 h at 37 °C and, after extensive washing with PBS, a biotinylated secondary mouse anti-human IFN-γ monoclonal antibody (0.05 μg ml −1 ; Mabtech) was added. The plates were developed using an alkaline phosphatase-conjugating substrate AP colour reagent A+B (BioRad). After 15 min, the colorimetric reaction was stopped by washing with tap water. Plates were air dried and spots were counted using an automated ELISpot reader (AID ELISpot Reader System). IFN-γ-producing T cells were expressed as spot-forming units per 1×10 6 cells. The number of specific IFN-γ-secreting cells was calculated by subtracting the unstimulated control value from the stimulated sample. Sequence evolution and bioinformatics software For sequence evaluation in evolutionary studies, PCR amplification of HIV env , followed by cloning and sequencing, was performed as previously described [56] . Analyses of evolution and site-specific selection were performed using BEAST [27] and CODEML [57] . CODEML was used to identify sites that have been subjected to positive selection using site-specific codon models. These models allow d N /d S to vary among sites, with values significantly above 1 indicating sites that had been under positive selection. We compared the fit of models M7 (which does not allow any sites to have a d N /d S of above 1) with M8 (which fits a class of sites with a d N /d S of above 1), using a likelihood ratio rest. The empirical Bayesian approach implemented by CODEML was used to identify codons under positive selection, using a cut-off of >90%. BEAST was used to model the evolution of the viral sequences through time, using the lognormal relaxed clock distribution to accommodate rate variation among branches. The multiple alignments contained 969 nucleotides. BEAST was run for 60 million steps, with the first 10% discarded as burn-in, and convergence was checked using Tracer. All analyses were repeated to ensure convergence. A preliminary BEAST analysis was performed that included the proviral sequence data, as these samples spanned a longer period of time than just the sequences obtained from plasma samples. The rate of evolution and effective population size were estimated from these time-structured sequences, and used in an analysis including only sequences obtained from plasma samples. Accession numbers: HIV-1 envelope sequences have been deposited in GenBank under accession numbers HQ241073–HQ241186. How to cite this article: Huang, K.-H.G. et al . B-cell depletion reveals a role for antibodies in the control of chronic HIV-1 infection. Nat. Commun. 1:102 doi: 10.1038/ncomms1100 (2010).